Poly(ADP-ribose) binding to Chk1 at stalled replication forks is required for S-phase checkpoint activation Damaged replication forks activate poly(ADP-ribose) polymerase 1 (PARP1), which catalyses poly(ADP-ribose) (PAR) formation; however, how PARP1 or poly(ADP-ribosyl)ation is involved in the S-phase checkpoint is unknown. Here we show that PAR, supplied by PARP1, interacts with Chk1 via a novel PAR-binding regulatory (PbR) motif in Chk1, independent of ATR and its activity. iPOND studies reveal that Chk1 associates readily with the unperturbed replication fork and that PAR is required for efficient retention of Chk1 and phosphorylated Chk1 at the fork. A PbR mutation, which disrupts PAR binding, but not the interaction with its partners Claspin or BRCA1, impairs Chk1 and the S-phase checkpoint activation, and mirrors Chk1 knockdown-induced hypersensitivity to fork poisoning. We find that long chains, but not short chains, of PAR stimulate Chk1 kinase activity. Collectively, we disclose a previously unrecognized mechanism of the S-phase checkpoint by PAR metabolism that modulates Chk1 activity at the replication fork. Cell cycle checkpoints sense DNA damage and execute cell cycle arrest through the modulation of the activity of cell cycle regulators. Ataxia-telangiectasia-mutated (ATM) and ataxia-telangiectasia-related (ATR) protein kinases are the central components of the major DNA damage checkpoints in vertebrates [1] , [2] . While the ATM pathway is activated in response to DNA double-strand breaks, the ATR pathway is induced by replication fork damage (for example, by hydroxyurea treatment (HU)) or single-strand breaks (SSBs) (for example, induced by ultraviolet light (UV)). At the stalled replication fork, the Rad17-RFC clamp loader recognizes the replication protein A (RPA)-coated ssDNA and assists with the loading of the Rad9–Hus1–Rad1 (9–1–1) complex [3] , which further recruits TopBP1. On one hand, TopBP1 activates ATR with help of ATRIP, while on the other hand, it bridges the 9–1–1 complex with checkpoint mediators (for example, Claspin) to present Chk1 to ATR [4] , [5] , [6] . Activated Chk1 phosphorylates its downstream substrate Cdc25a (refs 7 , 8 ), thus destabilizing it, to prevent the firing of later origins [9] . This process is essential in establishing the S-phase checkpoint to block replication fork progression, whereas deficiency of ATR or Chk1 abolishes this checkpoint and causes cellular and organismal lethality [10] , [11] , [12] , [13] , [14] , [15] , [16] , [17] . Although ATR and its upstream partners have been mapped to damaged replication forks, how Chk1 is activated by upstream kinases in the vicinity of these replication forks remains rather speculative. SSBs and replication poisons also activate poly(ADP-ribose) polymerase-1 (PARP1), which catalyses the synthesis of poly(ADP-ribose) polymers (PAR) and attaches them to target proteins [18] , whereas poly(ADP-ribose) glycohydrolase (PARG) rapidly hydrolyses PAR [19] , [20] . PARP1 is a known component of the base excision repair pathway [21] , [22] . Both Poly(ADP-ribosyl)ation and PARP1 have been shown to be important in multiple cellular processes, including DNA repair, proliferation, apoptosis, transcription, chromosomal stability and ageing [21] , [23] , [24] , [25] , [26] . More specifically, PARP1 modifies many target (‘acceptor’) proteins with large amounts of PAR. PARP1 and poly(ADP-ribosyl)ation have been suggested to regulate ATM or ATR activation in response to double-strand breaks and SSBs [27] , [28] , [29] . PAR is a highly negatively charged moiety and it has been hypothesized to be a signal to other cellular targets for recruitment to the damage sites [21] . However, the mechanisms by which targeted proteins sense the signal and are then located to the damage site remain poorly understood. Recently, huge effort has been devoted to the search for PAR-binding motifs in proteins to elucidate the biological function of PARPs and poly(ADP-ribosyl)ation. To date, three PAR-binding motifs have been identified in various proteins, including the putative consensus sequence of an eight amino-acid motif [30] , [31] , the PAR-binding zinc-finger (PBZ) motif [32] , [33] and the macrodomains [34] , [35] , [36] . Despite the universal nature of the poly(ADP-ribosyl)ation of target proteins, and PARP’s function in a wide range of cellular activities [21] , [25] , only a limited number of PAR-binding motifs have been found in several target proteins [20] , [37] . Therefore, the exploration of other PAR-binding motifs may help to understand the biological complexity of PAR metabolism in various cellular processes. Since the same type of DNA damage activates both PARP1 and the ATR–Chk1 pathway, and complete deletion of the PAR-forming (double knockout of PARP1 and PARP2 (ref. 38 )) or degrading enzymes ( PARG knockout [39] ) causes cellular and mouse lethality, similar to ATR- or Chk1-null mutations, we investigate whether these two processes are functionally linked and, if so, what the mechanism is. We report that the binding of PAR is required for Chk1 retention at damaged replication forks, and therefore full activation of the Chk1 kinase. The interaction occurs through a novel binding motif, the mutation of which impairs the S-phase checkpoint in vivo and renders cells hypersensitive to replication fork poisoning, at a similar level to Chk1 deficient cells, highlighting the fact that the homoeostasis of poly(ADP-ribosyl)ation is an essential function of Chk1 in response to replication damage. This finding uncovers a novel regulatory mechanism of the S-phase checkpoint. Hypo-poly(ADP-ribosyl)ation impairs the S-phase checkpoint We first tested, using a colony formation assay, whether altered PAR levels affected cell viability by SSBs and using replication fork poisons. In response to HU or the alkylating agent N -methyl- N ′-nitro- N -nitrosoguanidine (MNNG), PARP1 −/− mouse embryonic fibroblasts (MEFs) formed far fewer colonies when compared with wild-type controls ( Fig. 1a and Supplementary Fig. S1a,b ). As deletion of the PARG 110 isoform in MEF cells impairs turnover of the PAR-forming substrate and thus results in a very low amount of PAR [40] , we also found an intermediate, but significant, level of cytotoxicity in PARG 110 −/− cells compared with wild type and PARP1 −/− cells ( Fig. 1a and Supplementary Fig. S1a,b ). Notably, 2 mM HU significantly compromised colony formation in PARP1 −/− MEFs compared with wild-type cells (# P =0.0068, Student’s t -test), whereas high doses (>5 mM) of HU significantly reduced colony number in both PARP1 −/− and PARG 110 −/− cells compared with wild-type controls (* P <0.05, *** P <0.01, analysis of variance (ANOVA) test, Fig. 1a ). Cell survival appears to correlate with the cellular PAR level. 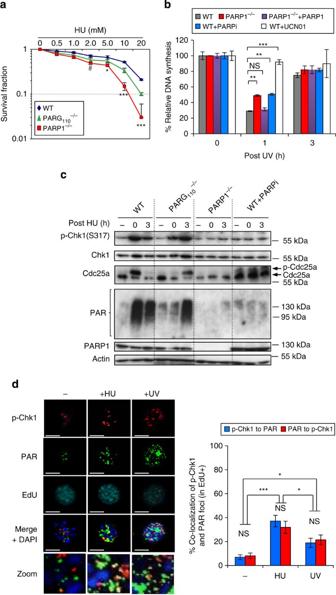Figure 1: S-phase defects after the inactivation of poly(ADP-ribosyl)ation. (a) Colony formation of 3T3 MEFs of wild type (WT),PARG110−/−andPARP1−/−genotype with or without HU treatment at the concentration indicated. The data represent the mean of two experiments using two independent cell lines from each genotype in duplicate. Error bars represent the s.e.m. Thet-test shows significant difference ofPARP1−/−cells as compared with WT cells (#P=0.0068). (b) RDS assay of immortalized MEFs of indicated genotype and treatment. Wild type (A19),PARP1−/−(A11),PARP1−/−reconstituted with human PARP1 cDNA (PARP1−/−+PARP1; A11/WT2), WT pretreated with the PARP inhibitor (PARPi, PJ-34, 10 μM) and WT cells pretreated with the Chk1 inhibitor UCN-01 (100 nM) at 2 h before UV treatment. The ratio of3H- (after) and14C- (before) labelled DNA was calculated after UV treatment (3 J m−2) and the relative DNA synthesis is shown. The data presented are the mean of two experiments using two independent cell lines from each genotype in triplicates. Error bars represent the s.e.m. (c) IB analysis of thymidine block-synchronized primary MEFs of indicated genotype wild type (WT),PARG110−/−,PARP1−/−and WT pre-incubated with the PARP inhibitor (PARPi, PJ-34, 10 μM) after treatment with 2 mM HU for 3 h. Untreated cells (−), or from 0 and 3 h after HU washout were analysed for the indicated proteins or PAR. Actin was used as a loading control. (d) Co-localization of PAR and p-Chk1 foci after both HU and UV damage. Representative images (left panel) and the quantification (right panel) of co-localization of PAR and phospho-Chk1 (p-Chk1) foci in EdU-positive MEF cells after HU (4 mM) or UV (10 J m−2) treatment. Insets show the enlarged image of co-localization of the PAR-p-Chk1 foci. Scale bar, 5 μm. For statistical evaluation, ANOVA followed by the Newman–Keulspost hocanalysis was performed. *P<0.05; **P<0.01; ***P<0.001. NS, not significant. Figure 1: S-phase defects after the inactivation of poly(ADP-ribosyl)ation. ( a ) Colony formation of 3T3 MEFs of wild type (WT), PARG 110 −/− and PARP1 −/− genotype with or without HU treatment at the concentration indicated. The data represent the mean of two experiments using two independent cell lines from each genotype in duplicate. Error bars represent the s.e.m. The t -test shows significant difference of PARP1 −/− cells as compared with WT cells (# P =0.0068). ( b ) RDS assay of immortalized MEFs of indicated genotype and treatment. Wild type (A19), PARP1 −/− (A11), PARP1 −/− reconstituted with human PARP1 cDNA ( PARP1 −/− +PARP1; A11/WT2), WT pretreated with the PARP inhibitor (PARPi, PJ-34, 10 μM) and WT cells pretreated with the Chk1 inhibitor UCN-01 (100 nM) at 2 h before UV treatment. The ratio of 3 H- (after) and 14 C- (before) labelled DNA was calculated after UV treatment (3 J m −2 ) and the relative DNA synthesis is shown. The data presented are the mean of two experiments using two independent cell lines from each genotype in triplicates. Error bars represent the s.e.m. ( c ) IB analysis of thymidine block-synchronized primary MEFs of indicated genotype wild type (WT), PARG 110 −/− , PARP1 −/− and WT pre-incubated with the PARP inhibitor (PARPi, PJ-34, 10 μM) after treatment with 2 mM HU for 3 h. Untreated cells (−), or from 0 and 3 h after HU washout were analysed for the indicated proteins or PAR. Actin was used as a loading control. ( d ) Co-localization of PAR and p-Chk1 foci after both HU and UV damage. Representative images (left panel) and the quantification (right panel) of co-localization of PAR and phospho-Chk1 (p-Chk1) foci in EdU-positive MEF cells after HU (4 mM) or UV (10 J m −2 ) treatment. Insets show the enlarged image of co-localization of the PAR-p-Chk1 foci. Scale bar, 5 μm. For statistical evaluation, ANOVA followed by the Newman–Keuls post hoc analysis was performed. * P <0.05; ** P <0.01; *** P <0.001. NS, not significant. Full size image The HU hypersensitivity of poly(ADP-ribosyl)ation-deficient cells prompted us to investigate whether PARP1 deficiency influences the S-phase checkpoint. To this end, we applied a radio-resistant DNA synthesis (RDS) assay [41] to measure replicative DNA synthesis after UV treatment. As expected, UV damage induced a strong intra-S-phase checkpoint in wild-type MEFs, judged through lower levels of DNA synthesis. In contrast, PARP1 −/− cells showed significantly higher DNA synthesis compared with wild-type cells ( P <0.01, ANOVA test). Reconstitution of PARP1 −/− cells with human PARP1 complementary DNA [42] could suppress this elevated DNA synthesis ( Fig. 1b ). Similar to PARP1-knockout cells, PARP inhibitor (PJ-34) treatment also resulted in a significantly higher amount of DNA synthesis when compared with wild-type cells ( Fig. 1b ). As a control, treatment of wild-type cells with the Chk1 inhibitor UCN-01 (ref. 43 ) relieved the UV-induced replication arrest ( P <0.001, ANOVA test, Fig. 1b ). These results indicate that inhibition of poly(ADP-ribosyl)ation compromises the intra-S-phase checkpoint, reminiscent of Chk1 inhibition-induced S-phase defects. To examine the molecular basis of the impaired S-phase checkpoints in poly(ADP-ribosyl)ation-deficient cells, double thymidine block-synchronized primary MEFs were treated with HU and analysed by immunoblotting. While HU-induced phosphorylation of Chk1 (p-Chk1), indicative of Chk1 activation, was readily visible in wild-type cells at 0 h after drug removal, this induction was abrogated in PARP1 −/− MEFs and in wild-type MEFs incubated with PARP inhibitor (PJ-34) ( Fig. 1c ). Moreover, a delayed p-Chk1 induction was found in hypo-poly(ADP-ribosyl)ated PARG 110 −/− cells (3 h, compared with 0 h post HU in wild-type MEFs; Fig. 1c ). Concomitantly, phosphorylation of the Chk1 downstream target Cdc25a was also impaired ( Fig. 1c ). We also found a reduction of p-RPA, a substrate of ATR, in PARP1 −/− cells and in wild-type cells treated with PARP inhibitor, compared with wild-type cells ( Supplementary Fig. S2 ), indicating that the PARP1 protein, but less probably PAR, plays a direct role in the ATR activation as suggested by a previous study [28] . However, ATM autophosphorylation was not evident after treatment with HU ( Supplementary Fig. S2 ), suggesting that replication poisoning does not activate ATM in this experimental setting [44] , [45] . Interestingly, immunoblotting with a PAR antibody revealed a correlation of the p-Chk1 level with the PAR pattern in these cells ( Fig. 1c ), suggesting that Chk1 activation behaviours may be due to the different capacities of these cells for poly(ADP-ribosyl)ation. Next, cell imaging analysis was performed to visualize the formation of PAR and p-Chk1 foci following UV or HU treatment. Since Chk1 activation is cell cycle dependent [46] , we quantified p-Chk1 foci only in S-phase cells, pre-labelled with 5-ethynyl-2-deoxyuridine (EdU). HU or UV treatment induced foci co-localization of PAR and p-Chk1 among EdU-positive cells, with a higher rate induced by HU as compared with UV treatment ( Fig. 1d ), suggesting a possible interaction of PAR and p-Chk1. As a control, knockdown of endogenous Chk1 by shChk1 ( Supplementary Fig. S3a ) greatly diminished the p-Chk1 foci ( Supplementary Fig. S3b,c ). PAR deficiency compromises the fork retention of Chk1 To further examine the spatio-temporal dynamics of Chk1 at the replication fork and its possible interaction with PARP1 or PAR, we applied the isolation of proteins on nascent DNA (iPOND) assay [47] , which allowed us to visualize Chk1 directly in the replication fork versus fork-free chromatin ( Fig. 2a ). First, we studied the kinetics of Chk1 protein distribution at the replication fork and also at fork-free chromatin (‘thymidine chase’) in HEK293 cells after HU treatment ( Fig. 2b ). The iPOND assay revealed that Chk1 was highly enriched in the replication fork fraction in comparison with the fork-free chromatin fraction in unchallenged or HU-treated cells ( Fig. 2b ). After HU treatment, the amount of Chk1 at the replication fork was reduced over time ( Fig. 2b ). Intriguingly, PARP inhibitor (AG014699) treatment resulted in significantly less Chk1 binding at the replication fork in HU-treated cells (* P <0.05, ** P <0.01, ANOVA test, Fig. 2c ). In addition, while a minor effect of Chk1 association was observed in unchallenged PARP1 −/− MEFs, Chk1 binding to the replication fork was greatly reduced in HU-treated PARP1 −/− MEFs compared with control MEFs ( PARP1 −/− reconstituted with PARP1 cDNA) (* P <0.05, ANOVA test, Fig. 2e ). Moreover, p-Chk1 was highly enriched at replication forks after HU treatment (1 h), but gradually reduced over time. At 4 h, the amount of p-Chk1-bound form at the replication fork was much lower in PARP1 −/− MEF cells compared with controls (* P <0.05, ANOVA test, Fig. 2e ). These data suggest that PAR may interact with and stabilize Chk1 at damaged forks. Of note, the binding of p-RPA to the replication fork was also induced after HU, but it was less in PARP1 −/− cells ( Fig. 2e ), possibly because of PARP1’s role in MRN-mediated resection at the replication fork that activates ATR [48] . Despite a great effort, all available PAR and PARP1 antibodies failed to visualize PAR and PARP1 binding at the replication fork, probably because of stringent technical requirement of this assay. 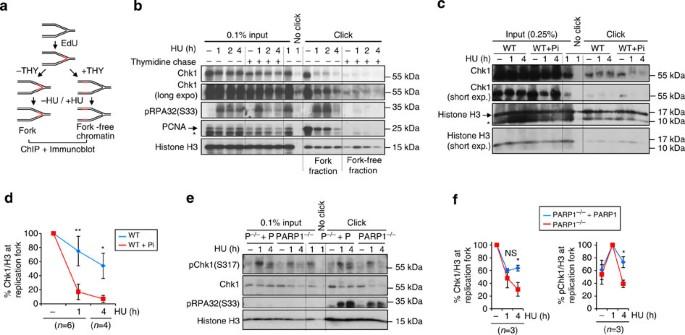Figure 2: The dynamics of PAR-dependent Chk1 association at the replication fork. (a) Schematic illustration of the iPOND assay. Cells were labelled with 10 μM EdU for 10 min, and then treated either without thymidine (−THY) to label the replication fork or chased with 10 μM thymidine (+THY) to label the fork-free chromatin, followed by treatment with 3 mM HU for the indicated times. Antibodies against the proteins of interest are used to perform the immunoblotting assay. (b) iPOND analysis of the replication fork associated proteins in HEK293 cells. Images of the western blot analysis of protein complexes from EdU-labelled DNA. PCNA was used to mark replication forks, while p-RPA indicates that checkpoint activation at the replication fork. (c) PAR influences Chk1 binding to the replication fork in HEK293 cells. Cells were pretreated with PARP inhibitor (AG014699, 1 μM) 1 h before the iPOND assay. (d) Quantification of the Chk1 bands normalized by H3 from duplicated samples of at least two independent experiments.n, the number of blots that were used for quantification. (e) iPOND analysis of replication fork associated proteins inPARP1−/−(A11) andPARP1−/−+ PARP1 (A11/WT2) (P−/−+P) MEF cells. (f) Quantification of Chk1 and p-Chk1 bands normalized by H3 from three blots of two independent experiments.n, the number of blots that were used for quantification. Input: the percentage of total protein; ‘no click’: unspecific protein binding to DNA precipitation beads; PCNA is a control for the replication fork fraction; p-RPA32(S33) control for activation of the S-phase checkpoint; histone H3 antibody control for loading of precipitated chromatin. Error bars represent the s.e.m. Figure 2: The dynamics of PAR-dependent Chk1 association at the replication fork. ( a ) Schematic illustration of the iPOND assay. Cells were labelled with 10 μM EdU for 10 min, and then treated either without thymidine (−THY) to label the replication fork or chased with 10 μM thymidine (+THY) to label the fork-free chromatin, followed by treatment with 3 mM HU for the indicated times. Antibodies against the proteins of interest are used to perform the immunoblotting assay. ( b ) iPOND analysis of the replication fork associated proteins in HEK293 cells. Images of the western blot analysis of protein complexes from EdU-labelled DNA. PCNA was used to mark replication forks, while p-RPA indicates that checkpoint activation at the replication fork. ( c ) PAR influences Chk1 binding to the replication fork in HEK293 cells. Cells were pretreated with PARP inhibitor (AG014699, 1 μM) 1 h before the iPOND assay. ( d ) Quantification of the Chk1 bands normalized by H3 from duplicated samples of at least two independent experiments. n , the number of blots that were used for quantification. ( e ) iPOND analysis of replication fork associated proteins in PARP1 −/− (A11) and PARP1 −/− + PARP1 (A11/WT2) (P −/− +P) MEF cells. ( f ) Quantification of Chk1 and p-Chk1 bands normalized by H3 from three blots of two independent experiments. n , the number of blots that were used for quantification. Input: the percentage of total protein; ‘no click’: unspecific protein binding to DNA precipitation beads; PCNA is a control for the replication fork fraction; p-RPA32(S33) control for activation of the S-phase checkpoint; histone H3 antibody control for loading of precipitated chromatin. Error bars represent the s.e.m. Full size image Interaction of PAR and Chk1 in vivo The iPOND results suggested that Chk1 interacts with PAR and PARP1. Therefore, we performed immunoprecipitation (IP) and immunoblot (IB) analysis to examine the relationship of PAR, PARP1 and Chk1. To preserve non-covalent PAR binding to Chk1, we used a native slot-blot assay. Following HU treatment, Chk1 and PAR antibodies precipitated a significant amount of PAR and Chk1, respectively, in wild-type MEF cell extracts ( Fig. 3a ). As a control, reciprocal IP using these antibodies pulled down a negligible amount of Chk1 or PAR either in wild-type cells treated with a PARP inhibitor or in PARP1 −/− cells ( Fig. 3a ). Reciprocal co-immunoprecipitation (Co-IP) by Chk1 and PARP1 antibodies also pulled down PARP1 and Chk1, respectively, in wild-type cells ( Fig. 3a ). However, PARP inhibitor treatment of wild-type cells (WT+PARPi) abolished PARP1-Chk1 binding ( Fig. 3a ), suggesting that PARP1 does not interact directly with Chk1, but via PAR. Of note, a basal level of IP products of both PARP1 and PAR was readily detectable in wild-type cells without HU treatment, which could nevertheless be inhibited by pretreatment with a PARP inhibitor ( Fig. 3a ). Furthermore, Chk1–PAR interaction was not mediated by DNA or chromatin because pretreatment of the cell lysates with DNase or ethidium bromide did not alter the amount of Chk1 pulled down by the PAR antibody (data not shown). 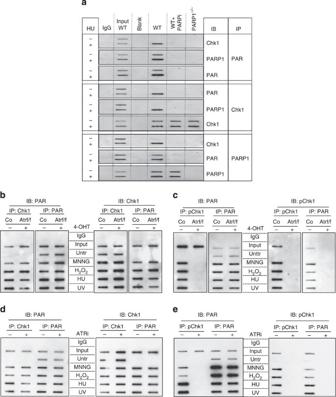Figure 3: Interaction of PAR and Chk1in vivois independent of Atr. (a) Co-immunoprecipitation (IP) and non-denaturing slot-blot analysis of PAR, Chk1 and PARP1 interaction in pMEFs from indicated genotype and treatment. pMEFs without (−) or with 2 mM HU treatment (3 h) were IP and immunoblotted (IB) using antibodies against PAR, Chk1 or PARP1. Ten percent of the cell lysates were used as inputs. (b,c) Co-IP and non-denaturing slot-blot analysis of the interaction between PAR and Chk1 (b), or between PAR and p-Chk1 (c) inAtrf/fMEFs cultured without 4-OHT (−) or with 4-OHT (+, 2 μM). The MEFs, which were untreated (Untr) or treated with MNNG (2 μM for 3 h), H2O2(10 μM for 30 min), 4 mM HU (3 h) or UV (100 J m−2), were IP and IB by antibodies against PAR, Chk1 or p-Chk1(S317). Ten percent of the cell lysates were used as Inputs. (d,e) Co-IP and non-denaturing slot-blot analysis of the interaction between PAR and Chk1 (d) or between PAR and p-Chk1 (e) in MEFs after DNA damage without (−) or with ATR inhibitor (ETP-46464, 10 μM) treatment for 2 h. The MEFs were untreated (Untr) or treated with MNNG (2 μM for 3 h), H2O2(10 μM for 30 min), 4 mM HU (3 h) or UV (100 J m−2) and followed by IP and IB by the antibody against PAR, Chk1 or p-Chk1(S317), respectively. Ten percent of the cell lysates were used as input. Figure 3: Interaction of PAR and Chk1 in vivo is independent of Atr. ( a ) Co-immunoprecipitation (IP) and non-denaturing slot-blot analysis of PAR, Chk1 and PARP1 interaction in pMEFs from indicated genotype and treatment. pMEFs without (−) or with 2 mM HU treatment (3 h) were IP and immunoblotted (IB) using antibodies against PAR, Chk1 or PARP1. Ten percent of the cell lysates were used as inputs. ( b , c ) Co-IP and non-denaturing slot-blot analysis of the interaction between PAR and Chk1 ( b ), or between PAR and p-Chk1 ( c ) in Atr f/f MEFs cultured without 4-OHT (−) or with 4-OHT (+, 2 μM). The MEFs, which were untreated (Untr) or treated with MNNG (2 μM for 3 h), H 2 O 2 (10 μM for 30 min), 4 mM HU (3 h) or UV (100 J m −2 ), were IP and IB by antibodies against PAR, Chk1 or p-Chk1(S317). Ten percent of the cell lysates were used as Inputs. ( d , e ) Co-IP and non-denaturing slot-blot analysis of the interaction between PAR and Chk1 ( d ) or between PAR and p-Chk1 ( e ) in MEFs after DNA damage without (−) or with ATR inhibitor (ETP-46464, 10 μM) treatment for 2 h. The MEFs were untreated (Untr) or treated with MNNG (2 μM for 3 h), H 2 O 2 (10 μM for 30 min), 4 mM HU (3 h) or UV (100 J m −2 ) and followed by IP and IB by the antibody against PAR, Chk1 or p-Chk1(S317), respectively. Ten percent of the cell lysates were used as input. Full size image Interaction of PAR and Chk1 can be Atr-independent Although PAR forms in response to DNA damage [21] , [25] , [26] , many DNA-damaging treatments, in particular alkylating agents, can induce PAR rapidly, without activating ATR, until the DNA lesion is processed. This caused us to ask whether Chk1–PAR binding is a general phenomenon after DNA damage. Co-IP-IB and native slot-blot assays revealed that the treatment of cells with various DNA damage agents, regardless of whether they damage chromatin DNA (MNNG, H 2 O 2 , UV) or replication forks (HU), resulted in Chk1–PAR interaction ( Fig. 3b ). To test whether the interaction is dependent on ATR activation, we established floxed Atr (Atr- CreER T2 ) MEFs, in which Atr deletion is inducible by the addition of 4-hydroxy tamoxifen (4-OHT) in culture ( Supplementary Fig. S4 ) and challenged these cells with various DNA damage agents. Apparently, the interaction of PAR and Chk1 was unaffected after Atr deletion ( Fig. 3b ), whereas the interaction of PAR and p-Chk1 was diminished in Atr-deleted cells ( Fig. 3c ), which is consistent with the dependence of Chk1 phosphorylation on Atr. To further test whether the Atr protein per se is necessary for Chk1–PAR interaction, we applied an ATR inhibitor [49] . Similar to Atr -knockout cells, the ATR inhibitor had a minor, if any, effect on PAR–Chk1 interaction ( Fig. 3d ). As expected, the ATR inhibitor diminished the binding of PAR with p-Chk1 ( Fig. 3e ). Thus, these results indicate that PAR interacts with both Chk1 and p-Chk1, raising the possibility that Chk1 can be phosphorylated in a PAR-bound form. These results, together with the iPOND data ( Fig. 2b–f ) suggest that interaction of Chk1 and PAR is a general DNA damage response in both chromatin and replication forks but can occur independently from the Chk1 upstream kinase ATR. PAR binding may retain and facilitate the phosphorylation of Chk1 by upstream kinases, such as ATR, at the vicinity of damaged replication forks. Identification of the PAR-binding motif in Chk1 To further test whether PAR can interact directly with Chk1, and not through a third partner in vivo , we performed an in vitro PAR-binding (dot-blot) assay. We blotted glutathione S -transferase (GST)-tagged wild-type Chk1 (GST-wtChk1) proteins ( Supplementary Fig. S5a ) onto a nitrocellulose membrane and incubated with radiolabelled PAR ( 32 P-PAR). Autoradiography of the blots revealed a strong PAR binding with GST-wtChk1 ( Fig. 4a ). The binding capacity/efficiency was similar to that of positive control histones H1 and H4 (refs 50 , 51 ). The binding appeared to be stable as the signal was maintained after a stringent TBS-T washing (600 mM NaCl) ( Fig. 4a ). In addition, washing of the blots with 20 mM EDTA had a minor effect on the binding of PAR to Chk1 ( Fig. 4a ), indicating that metal ions are unlikely to have a major impact on the binding. 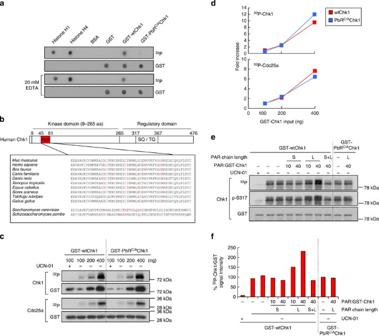Figure 4: Chk1 binds to PAR via the PbR motif and facilitates its kinase activity. (a) Dot-blot assay of PAR binding of Chk1. Indicated protein (1 pmol) was spotted onto a nitrocellulose membrane and incubated with32P-labelled PAR. The blots were washed with TBS-T buffer containing 600 mM NaCl plus 20 mM EDTA (lower panels). PAR-bound proteins were then visualized by autoradiography. Positive controls (Histone H1 and H4) and negative controls (BSA and GST) were included. Loading of GST-tagged proteins was confirmed by staining with an anti-GST antibody. (b) Identification of the putative PAR-binding motif in Chk1. A putative PAR-binding motif in Chk1 and was designated the ‘PAR-binding regulatory (PbR) motif’. Note that the PbR site (indicated in red) is highly conserved among vertebrates but not in yeast. (c) Chk1 kinase activity assay. GST-tagged wild-type Chk1 (GST-wtChk1) or PbR-mutant Chk1 (GST-PbRC/AChk1) proteins were incubated with 2 μg of GST-Cdc25a and [γ-32P]-ATP.32P incorporation was detected by autoradiography. GST-tagged protein was detected by an anti-GST antibody. The Chk1 inhibitor UCN-01 was added to 100 ng GST-Chk1 as a control. (d) The kinase activity is measured by32P incorporation in Chk1 or Cdc25a normalized for signal intensity of 100 ng wtChk1 input (GST signal) (c). (e) The kinase reaction was performed using recombinant GST-wtChk1 or GST-PbRC/AChk1 (100 ng). These proteins were incubated with size-fractionated PAR (S: 26–30 units; L: >65 units; S+L: 1:1 mixture of short- and long-chain PAR). PAR:GST-Chk1: molar ratio of (ADP-ribose) units within the PAR polymer to GST-Chk1 molecules, 10 or 40, respectively. The amount of ADP ribose units and thus negative charges are similar in the reactions with either long or short PAR polymer.32P incorporation was detected by autoradiography. GST-tagged protein was detected by an anti-GST antibody. Phospho-Chk1 was blotted by a specific antibody against p-Chk1(S317). The Chk1 inhibitor UCN-01 was used as a control. The asterisk indicates an unspecific band. (f) Quantification of32P incorporation in Chk1 is shown in panele. Figure 4: Chk1 binds to PAR via the PbR motif and facilitates its kinase activity. ( a ) Dot-blot assay of PAR binding of Chk1. Indicated protein (1 pmol) was spotted onto a nitrocellulose membrane and incubated with 32 P-labelled PAR. The blots were washed with TBS-T buffer containing 600 mM NaCl plus 20 mM EDTA (lower panels). PAR-bound proteins were then visualized by autoradiography. Positive controls (Histone H1 and H4) and negative controls (BSA and GST) were included. Loading of GST-tagged proteins was confirmed by staining with an anti-GST antibody. ( b ) Identification of the putative PAR-binding motif in Chk1. A putative PAR-binding motif in Chk1 and was designated the ‘PAR-binding regulatory (PbR) motif’. Note that the PbR site (indicated in red) is highly conserved among vertebrates but not in yeast. ( c ) Chk1 kinase activity assay. GST-tagged wild-type Chk1 (GST-wtChk1) or PbR-mutant Chk1 (GST-PbR C/A Chk1) proteins were incubated with 2 μg of GST-Cdc25a and [γ- 32 P]-ATP. 32 P incorporation was detected by autoradiography. GST-tagged protein was detected by an anti-GST antibody. The Chk1 inhibitor UCN-01 was added to 100 ng GST-Chk1 as a control. ( d ) The kinase activity is measured by 32 P incorporation in Chk1 or Cdc25a normalized for signal intensity of 100 ng wtChk1 input (GST signal) ( c ). ( e ) The kinase reaction was performed using recombinant GST-wtChk1 or GST-PbR C/A Chk1 (100 ng). These proteins were incubated with size-fractionated PAR (S: 26–30 units; L: >65 units; S+L: 1:1 mixture of short- and long-chain PAR). PAR:GST-Chk1: molar ratio of (ADP-ribose) units within the PAR polymer to GST-Chk1 molecules, 10 or 40, respectively. The amount of ADP ribose units and thus negative charges are similar in the reactions with either long or short PAR polymer. 32 P incorporation was detected by autoradiography. GST-tagged protein was detected by an anti-GST antibody. Phospho-Chk1 was blotted by a specific antibody against p-Chk1(S317). The Chk1 inhibitor UCN-01 was used as a control. The asterisk indicates an unspecific band. ( f ) Quantification of 32 P incorporation in Chk1 is shown in panel e . Full size image The interaction data from in vivo Co-IP experiments and the in vitro dot-blot assay prompted us to search for potential PAR-binding motifs in Chk1. On the basis of all known PAR-binding motifs or domains, such as the PBZ motif [32] , eight amino-acid motif [30] and macrodomains [34] , [35] , [36] , we blasted the databases (Ensembl; http://www.ensembl.org/index.html , RCSB Protein Data Bank http://www.pdb.org/pdb/home/home.do and ExPASy http://www.expasy.org/ ) but did not find any of these motifs in Chk1. However, we detected a putative C2H2 motif (C 8 -C 6 -H 8 -H) in the amino terminus of Chk1, which is distinct from the canonical PBZ C2H2 (C 8 -C 8 -H 8 -H) but displays a strong regularity of amino-acid sequences ( Fig. 4b ). Intriguingly, this motif is highly conserved among vertebrate species ( Fig. 4b ), but not in yeast, an organism that lacks PARPs and poly(ADP-ribosyl)ation. These findings argue that this sequence may well serve as a functional PAR-binding motif, which we have designated ‘PAR-binding regulatory (PbR) motif’. PAR binding of Chk1 modulates its kinase activity We next investigated the biochemical properties of the PbR motif. As the PbR motif is located in the kinase domain, we first verified whether any mutations introduced into the PbR motif would interfere with the Chk1 kinase activity. To this end, we performed an in vitro assay using purified GST-tagged wtChk1 and PbR C/A Chk1 proteins. We found that these two proteins harboured a similar kinase activity, as judged by the autophosphorylation of Chk1 and the phosphorylation of its downstream target Cdc25a ( Fig. 4c ), confirming that point mutations introduced into the PbR motif do not affect Chk1’s intrinsic kinase activity. To test whether the PAR binding by Chk1 is indeed via PbR, we performed the PAR-binding dot-blot assay using purified GST-tagged PbR-mutant Chk1 proteins, in which the PbR site was mutated by replacing two cysteines with alanines (Chk1 C48A/C57A ; GST-PbR C/A Chk1). In contrast to the GST-wtChk1, autoradiograph of the blots revealed no PAR binding with GST-PbR C/A Chk1 ( Fig. 4a ), thus demonstrating that the PbR motif is responsible for PAR interaction with Chk1. It is known that the non-covalent binding of proteins to PAR can influence their functionality [52] . We then investigated the impact of PAR binding to Chk1 on the protein’s kinase activity. We incubated GST-wtChk1 or GST-PbR C/A Chk1 with PAR of different lengths ( Supplementary Fig. S5b ) and at various ratios, and then performed the in vitro kinase activity assay using Chk1 autophosphorylation at S317 as the read-out [53] . When GST-wtChk1 was incubated with short-chain PAR (26–30 moieties), Chk1 phosphorylation was unchanged compared with controls without PAR ( Fig. 4e ). However, long-chain PAR (>65 moieties) stimulated wtChk1 autophosphorylation, indicative of Chk1 activity, but failed to do so with the PbR-mutant Chk1, even after the amount of PAR was doubled ( Fig. 4e ; see also Supplementary Fig. S5c,d ). Intriguingly, when short-chain PAR and long-chain PAR were combined, the stimulating effect of long PAR chains on Chk1 kinase activity was repressed ( Fig. 4e ). To test whether PARP1 itself would be sufficient to activate Chk1 kinase activity, we performed an in vitro kinase activity assay for Chk1. We first synthesized PAR in vitro by incubating PARP1 with NAD + together with activated DNA. After adding Chk1, its kinase activity was measured ( Supplementary Fig. S5d ). We found that just the PARP1 protein itself (either without NAD+ or addition of PARP inhibitor) was unable to activate Chk1, and only poly(ADP-ribosyl)ated PARP1 could stimulate Chk1 phosphorylation ( Supplementary Fig. S5d ). Notably, activated DNA alone did not stimulate Chk1 activity, indicating that the stimulatory effect was specific to PAR and not general to any negatively charged polymers. Together with the Co-IP-IB data ( Fig. 3a ), we conclude that PAR is a cofactor for Chk1 activation. The PbR motif mediates in vivo interaction of PAR and Chk1 To further confirm whether this PbR-mediated PAR–Chk1 interaction in vitro also occurs in vivo , we transfected Flag-tagged wild-type Chk1 (Flag-wtChk1) or mutant Chk1 (Flag-PbR C/A Chk1) constructs into U2OS cells. We performed Co-IP-IB in the native slot-blot assay using Flag (to detect Chk1), PAR or PARP1 antibodies. Consistent with the endogenous situation, we found Flag-wtChk1 interacted with PAR and PARP1 after HU treatment. However, these interactions were abolished when PbR was mutated in Chk1 ( Fig. 5a ). Taken together, binding of PAR to Chk1 is indeed mediated through the PbR motif. 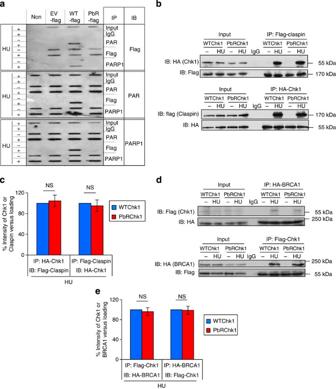Figure 5: The interaction of Chk1 with PAR and its canonical partners Claspin and BRCA1. (a) Co-IP and non-denaturing slot-blot analysis of PAR, Chk1 and PARP1 interaction in U2OS cells transfected with mock (Non), Flag-tagged empty vector (Flag-EV), wild-type Chk1 (Flag-wtChk1), and PbR-mutant Chk1 (Flag-PbRC/AChk1) and treated with or without HU (2 mM) for 3 h. Cell extracts at 0 h after HU removal were IP and IB by antibodies against Flag (for Chk1), PAR or PARP1. Ten percent of the cell lysates were used as an input. (b–e) The PbR mutation does not interfere with the interaction of Chk1 with Claspin or BRCA1. (b,d) Co-IP of Chk1-Claspin and Chk1-BRCA1. HEK293 cells were transfected with HA-Chk1 and Flag-Claspin (b), or Flag-Chk1 and HA-BRCA1 (d) and treated with or without HU (4 mM) for 3 h. Cell extracts at 0 h after HU removal were IP and IB by the antibodies against Flag- and HA-tag as indicated. (c,e) Quantifications of the signal intensity of the indicated proteins after normalization by respective loading (IB with HA or Flag in lower panels of each IPs) from three samples of two independent experiments. NS, not significant. Error bars represent the s.e.m. Figure 5: The interaction of Chk1 with PAR and its canonical partners Claspin and BRCA1. ( a ) Co-IP and non-denaturing slot-blot analysis of PAR, Chk1 and PARP1 interaction in U2OS cells transfected with mock (Non), Flag-tagged empty vector (Flag-EV), wild-type Chk1 (Flag-wtChk1), and PbR-mutant Chk1 (Flag-PbR C/A Chk1) and treated with or without HU (2 mM) for 3 h. Cell extracts at 0 h after HU removal were IP and IB by antibodies against Flag (for Chk1), PAR or PARP1. Ten percent of the cell lysates were used as an input. ( b – e ) The PbR mutation does not interfere with the interaction of Chk1 with Claspin or BRCA1. ( b , d ) Co-IP of Chk1-Claspin and Chk1-BRCA1. HEK293 cells were transfected with HA-Chk1 and Flag-Claspin ( b ), or Flag-Chk1 and HA-BRCA1 ( d ) and treated with or without HU (4 mM) for 3 h. Cell extracts at 0 h after HU removal were IP and IB by the antibodies against Flag- and HA-tag as indicated. ( c , e ) Quantifications of the signal intensity of the indicated proteins after normalization by respective loading (IB with HA or Flag in lower panels of each IPs) from three samples of two independent experiments. NS, not significant. Error bars represent the s.e.m. Full size image We next tested whether the PbR mutation would affect the Chk1 interaction with its partners in the ATR pathway [13] . First, we co-transfected haemagglutinin (HA)-tagged wild-type (HA-wtChk1) or PbR-mutant Chk1 (HA-PbR C/A Chk1) with Flag-Claspin and performed the Co-IP-IB assay. We found that both the wild-type and PbR-mutant Chk1 interacted equally well with Claspin ( Fig. 5b ). We also tested the interaction of PbR C/A Chk1 and BRCA1 and found normal interaction between PbR C/A Chk1 and BRCA1 ( Fig. 5d ). These data suggest that the PbR mutation does not affect the interaction of Chk1 with its activation mediators of the canonical ATR pathway. PbR mutation impairs Chk1-mediated S-phase checkpoint To study the biological effect of the PbR motif in HU-induced S-phase checkpoint, we engineered stable COS7 cell lines by ectopically expressing green fluorescent protein (GFP)-tagged empty vector (EV-GFP), wild-type Chk1 (wtChk1-GFP) or PbR-mutant Chk1 (PbR C/A Chk1-GFP) of mouse species ( Fig. 6a ). COS7 cells were chosen because we wanted to specifically knockdown the monkey Chk1 in these cells to minimize the influence of endogenous Chk1. To this end, we identified short interfering RNA (siRNA; siChk1-1 and siChk1-3) to knock down efficiently endogenous monkey Chk1 in these transfectants without interference of ectopically expressed wtChk1-GFP and PbR C/A Chk1-GFP (see Supplementary Fig. S6a,b ). Immunoblotting confirmed that the ectopic Chk1-GFP expression was similar in both wtChk1-GFP- and PbR C/A Chk1-GFP-infected cells ( Fig. 6b , top panel). We then analysed Chk1 activation in these cells after HU treatment. As expected, EV-GFP-transfected cells showed no detectable p-Chk1 and p-Cdc25a signals after endogenous Chk1 knockdown (siChk1) ( Fig. 6b ). While phosphorylation of wtChk1-GFP (p-Chk1) was evident at 0 h after HU treatment, this induction was greatly attenuated in PbR C/A Chk1-GFP-transfected cells ( Fig. 6b ). Consistent with the low levels of p-Chk1, phosphorylation of Cdc25a (p-Cdc25a) was also abrogated at 0 h after HU removal in PbR C/A Chk1-GFP-transfectants as compared with wtChk1-GFP-transfected cells ( Fig. 6b ). PbR C/A Chk1-GFP-transfected cells showed a similar pattern of p-RPA compared with wtChk1-GFP transfections ( Fig. 6b ), suggesting that the PbR mutation did not interfere with the upstream ATR pathway. Of note, we consistently found a constant p-RPA in siChk1-transfected cells ( Fig. 6b ), but for currently unknown reasons. 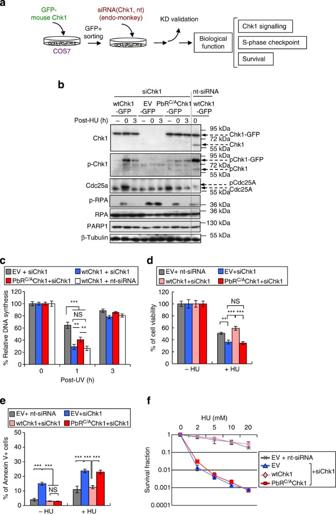Figure 6: Biological consequence of the PbR mutation in response to replication fork stress. (a) The experimental design to test the function of PbR. GFP-tagged Chk1 vectors were transfected into monkey COS7 cells. Endogenous monkey Chk1 is knocked down (KD) by monkey-specific siRNA. (b) IB analysis of Chk1 activation. COS7 cells stably transfected with empty vector-GFP (EV-GFP), wild type (wtChk1-GFP) or PbR-mutant Chk1 (PbRC/AChk1-GFP) vectors were treated with siChk1 or non-target siRNA (nt-siRNA). At 3 days after siRNA treatment, cells untreated (−) or treated with 2 mM HU for 3 h were analysed for the indicated proteins at 0 and 3 h after HU removal. COS7 cells (wtChk1-GFP+nt-siRNA) were used as controls. PARP1 and β-tubulin were used as loading controls. (c) RDS assay of COS7 cells transfected with indicated vectors after siChk1 or nt-siRNA treatment. The ratio of3H- (after) and14C- (before) labelled DNA was calculated after 3 J m−2UV treatment and the relative DNA synthesis is shown. The data are the mean of two experiments using two cell lines from each genotype in triplicates. Error bars represent the s.e.m. (d) Cell viability of COS7 cells stably expressing indicated vectors after depletion of endogenous Chk1 and treatment with 1.25 mM HU for 20 h. Cell numbers relative to untreated controls were quantified by high-content analysis microscopy. The data represent the mean of three independent experiments from each genotype in triplicate. Error bars represent the s.e.m. (e) Flow cytometric analysis of cells treated with 1.25 mM HU for 48 h. The Annexin V- and GFP-double-positive population was plotted. The data represent the mean of two independent experiments from each genotype in duplicate. Error bars represent the s.e.m. (f) Colony formation and dose-response of cells with indicated genotype and treatment. Data shown are one of two experiments. For statistical evaluation, ANOVA followed by Tukeypost hocanalysis was performed. **P<0.01; ***P<0.001. NS, not significant. Figure 6: Biological consequence of the PbR mutation in response to replication fork stress. ( a ) The experimental design to test the function of PbR. GFP-tagged Chk1 vectors were transfected into monkey COS7 cells. Endogenous monkey Chk1 is knocked down (KD) by monkey-specific siRNA. ( b ) IB analysis of Chk1 activation. COS7 cells stably transfected with empty vector-GFP (EV-GFP), wild type (wtChk1-GFP) or PbR-mutant Chk1 (PbR C/A Chk1-GFP) vectors were treated with siChk1 or non-target siRNA (nt-siRNA). At 3 days after siRNA treatment, cells untreated (−) or treated with 2 mM HU for 3 h were analysed for the indicated proteins at 0 and 3 h after HU removal. COS7 cells (wtChk1-GFP+nt-siRNA) were used as controls. PARP1 and β-tubulin were used as loading controls. ( c ) RDS assay of COS7 cells transfected with indicated vectors after siChk1 or nt-siRNA treatment. The ratio of 3 H- (after) and 14 C- (before) labelled DNA was calculated after 3 J m −2 UV treatment and the relative DNA synthesis is shown. The data are the mean of two experiments using two cell lines from each genotype in triplicates. Error bars represent the s.e.m. ( d ) Cell viability of COS7 cells stably expressing indicated vectors after depletion of endogenous Chk1 and treatment with 1.25 mM HU for 20 h. Cell numbers relative to untreated controls were quantified by high-content analysis microscopy. The data represent the mean of three independent experiments from each genotype in triplicate. Error bars represent the s.e.m. ( e ) Flow cytometric analysis of cells treated with 1.25 mM HU for 48 h. The Annexin V- and GFP-double-positive population was plotted. The data represent the mean of two independent experiments from each genotype in duplicate. Error bars represent the s.e.m. ( f ) Colony formation and dose-response of cells with indicated genotype and treatment. Data shown are one of two experiments. For statistical evaluation, ANOVA followed by Tukey post hoc analysis was performed. ** P <0.01; *** P <0.001. NS, not significant. Full size image We next examined the intra-S-phase checkpoint in these cells using the RDS assay. While wtChk1-GFP-expressing cells transfected with non-targeting siRNA (nt-siRNA) showed a repression of DNA synthesis after UV treatment, as expected, Chk1 knockdown in the EV-GFP-transfected cells alleviated this repression ( Fig. 6c ). Compared with wtChk1-GFP, PbR C/A Chk1-GFP had a significantly lower capacity to restore DNA synthesis repression in siChk1-transfected cells ( Fig. 6c ), indicating that PbR-mutant Chk1 renders cells to an intra-S-phase checkpoint defect. Therefore, cells expressing PbR-mutant Chk1 phenocopied PAR-deficient cells in their Chk1-mediated S-phase checkpoint signalling. PbR-mutant Chk1 confers a hypersensitivity to fork poisoning We next analysed the biological significance of the PbR motif using PbR-mutant Chk1-transfected cells. In a short-term cell survival assay, HU treatment resulted in significantly lower cell numbers in siChk1-treated COS7 cells (EV+siChk1), compared with control cells (EV+nt-siRNA; Fig. 6d ). While wtChk1 expression alleviated cell loss caused by siChk1, expression of PbR C/A Chk1 failed to do so, and cell survival was similar to siChk1-knockdown cells (EV+siChk1; Fig. 6d ). Consistently, Annexin V staining after 48 h treatment with HU revealed 24% cell death when endogenous Chk1 was knocked down (EV+siChk1) in contrast to 11% in nt-siRNA-treated control cells ( Fig. 6e ). This defect could be corrected by ectopic expression of wtChk1 but not of PbR-mutant Chk1 ( Fig. 6e ). It is interesting to note that exclusive expression of PbR C/A Chk1 could repress the spontaneous cell death of Chk1-knockdown cells (PbR C/A Chk1+siChk1) as efficiently as wtChk1 (wtChk1+siChk1) in the unchallenged condition ( Fig. 6e and Supplementary Fig. S7 ). Intriguingly, a long-term cell survival assay (colony formation) revealed severe cell lethality in response to HU treatment. As expected, siChk1 knockdown in EV-infected cells resulted in the formation of very few colonies after HU treatment ( Fig. 6f and Supplementary Fig. S7 ). This defect was fully corrected in cells ectopically expressing wtChk1. Strikingly, PbR C/A Chk1 expression in siChk1-treated cells could not rescue HU-induced cell loss, as only very few colonies formed, at a similar level to that of EV-transfected siChk1 cells ( Fig. 6f and Supplementary Fig. S7 ). Taken together, these findings indicate that PAR binding to Chk1 is essential for cell survival in response to replication stress but seems to be dispensable in the unchallenged condition. Recent studies have shown that domain-specific binding to PAR regulates the function of target proteins (see reviews by refs 20 , 37 ). PAR binds to the PBZ motif of APLF and CHFR to regulate the cellular response to DNA damage [32] , while PAR binding to the macrodomain of macroH2A1.1 controls chromatin remodelling [34] , [36] . These target-specific PAR-binding sites provide a diversity in regulatory mechanisms and highlight the importance of poly(ADP-ribosyl)ation in multiple cellular processes. In the present study, we have identified a novel PAR-binding site in the key checkpoint kinase Chk1, termed PbR motif. Interestingly, the PbR motif sequence is highly conserved in most vertebrate species, but not in yeast, which coincides with the fact that yeasts do not have PARPs, that is, they are devoid of poly(ADP-ribosyl)ation. Blasting of the PbR motif on several databases did not reveal any significant alignment with other proteins. Thus, PAR-mediated Chk1 regulation through PbR may have evolved in higher organisms harbouring PAR metabolism, allowing for a sophisticated regulatory mechanism of cell cycle control, via Chk1, to cope with replication damage and SSBs. It is generally believed that Chk1 is recruited to and activated at damaged replication forks [9] , [16] . However, the behaviour of Chk1 in undisturbed or damaged replication forks has not been formally documented. We found that Chk1 interaction with PAR is a general phenomenon in DNA lesions in both chromatin and replication forks. Interestingly, the inhibition of ATR activity or ATR deletion had a minor, if any, effect on the interaction of Chk1–PAR. Our iPOND experiments demonstrate for the first time that Chk1 is readily associated with unperturbed replication forks, which is in contrast to the general view that Chk1 is recruited to the stalled replication fork. We also observed that, after HU treatment, Chk1 falls off from the stalled replication fork, which is consistent with the notion that Chk1 disappears from chromatin after DNA damage [54] , [55] . Notably, Chk1 binding is more highly enriched at the undisturbed replication fork than that at non-fork chromatin. Although we cannot distinguish quantitatively the fraction of total Chk1 in chromatin versus the replication fork, Chk1 seems to preferentially bind at the replication fork. Importantly, PAR deficiency ( PARP1 −/− cells and PARP inhibitor treatment) attenuated Chk1 and p-Chk1 retention at the replication fork after replication poisoning ( Fig. 2c–f ). Interestingly, PARP1 per se does not necessarily interact directly with Chk1. Together with the co-localization data ( Fig. 1d ), these results favour the idea that PAR interacts and stabilizes Chk1, facilitating its phosphorylation, and opening up the possibility that other poly(ADP-ribosyl)ated proteins may also interact with Chk1 via PAR in the proximity of the damaged fork. It is well documented that the phosphorylation of serines by kinases or the exchange of some amino acids in the carboxy terminal SQ/TQ domain switches on the kinase activity of Chk1 (refs 1 , 16 , 56 ). However, modifications of the N terminus that would modulate Chk1 activity have not yet been reported. A previous study [57] implied a hypothetical trans-regulatory molecule that can activate Chk1 activity, independent of phosphorylation of p-Chk1(S345) and of the C terminus. Our study identifies that the PbR motif in the N terminus of Chk1 does indeed stimulate its kinase activity after PAR binding. Intriguingly, the binding of Chk1 to a long PAR chain enhances its kinase activity. Although we do not know the nature of the stimulating activity by long chains of PAR, it is possible that a long chain or high local concentration of PAR acts as a scaffold to increase the availability and the spatial proximity of Chk1 for phosphorylation by upstream kinases, or itself. The fact that short-chain PARs lacked the stimulatory function and even repressed the stimulatory effect of long-chain PAR on Chk1 activation suggests the homeostasis of PAR in a regulatory mechanism of Chk1 activity. It is possible that the selective activation capacity by different sizes of PAR may also be a target-specific activation mechanism by which Chk1 only ‘talks’ to partners carrying certain PAR lengths. We speculate that this ‘on-off’ mode of Chk1 activation may strengthen a sensitive regulation of the Chk1-mediated checkpoint at which cells must decide quickly whether to halt or restart DNA replication. Nevertheless, how PAR chains (long, short or branched) can stimulate Chk1 kinase activity requires further structural-functional studies. PAR deficiency compromises the Chk1 retention at the replication fork and impairs Chk1 activation. We also observed less p-RPA in the iPOND assay ( Fig. 2e ) and in immunoblotting of PARP1 −/− cells ( Supplementary Fig. S2 ). As PARP1 is required for the recruitment of the MRN complex to resect DNA at the stalled replication forks [58] , [59] , the impaired activation of Chk1 in PAR-deficient conditions might be due to the decreased resection at stalled forks, leading to less RPA-ATR-Chk1 activation. However, since ATR is dispensable for Chk1–PAR binding and Chk1 is enriched at the replication fork without HU treatment, less p-RPA after damage is unlikely to contribute significantly to the accelerated dissociation of Chk1 from the replication fork. Moreover, PbR C/A Chk1-reconstituted cells in the PARP1-proficient background showed a similar S-phase checkpoint failure as PARP-deficient cells. Finally, although the PbR mutation compromised Chk1 activation, it did not interfere with the interaction with authentic partners (Claspin or BRCA1) of the canonical ATR pathway in response to replication stress, which uncouples PAR binding from the canonical ATR pathway. This also suggests that the impaired Chk1-mediated S-phase checkpoint is likely due to the impaired binding of PAR, but not the canonical ATR pathway. Altogether, we can conclude that the initial PAR binding by Chk1 is either parallel or upstream of Chk1 upstream kinases. Despite a relatively modest impact of the PbR mutation on the S-phase checkpoint after HU treatment ( Fig. 6c ), PbR-mutant Chk1 rendered cells hypersensitive to HU-induced cytotoxicity, at a level similar to that of Chk1-knockdown cells in the colony formation assay. This finding indicates that the loss of PAR binding is analogous to the loss-of-function of Chk1 in response to fork damage. Strikingly, unlike a null mutation, PbR-mutant Chk1 can repress spontaneous cell death in siChk1-knockdown cells without replication stress (see Fig. 6e ). Therefore, the PbR motif decouples the cell survival function of Chk1 in unperturbed proliferation from the replication poison-induced S-phase checkpoint. Both Chk1 and PARP inhibitors have been developed as drugs to treat human cancers [60] , [61] , [62] . Our study highlights PAR metabolism intervention in the PAR–Chk1 interaction as a potential strategy for the treatment of human malignancies. Our results demonstrate that PAR binding to Chk1 is an obligatory event during replication fork damage and contributes to the fine-tuning of the S-phase checkpoint imposed by Chk1. Here we propose a working model on how PAR is involved in the Chk1-mediated S-phase checkpoint (see Fig. 7 ). Via a currently unknown mechanism, Chk1 associates readily with an unperturbed replication fork. In response to a replication fork stall, PARP1 binds to replication forks [58] , [63] to catalyse PAR formation onto itself (as a major poly(ADP-ribosyl)ation acceptor) or other proteins. The pre-existing replication fork-bound Chk1 interacts with PAR via the PbR motif, independent of the ATR pathway. The PAR binding stabilizes Chk1 at the replication fork. In parallel, ATR, along with the help of ATRIP is recruited to and activated (later) by the upstream S-phase checkpoint complex at the stalled replication fork [13] . In the vicinity of PAR-bound Chk1, on association with its mediators, such as Claspin, ATR phosphorylates the C-terminal tails of Chk1. This is supported by the observation that p-Chk1 association to the replication fork is also attenuated if PAR is depleted ( Fig. 2e ). Finally, activated Chk1 is released from stalled replication forks to exert its checkpoint function ( Fig. 7 ). Whether the fall off of Chk1 (and p-Chk1) is assisted by the transient nature of PAR formation/degradation, or by high negative charges of PAR, which repels from DNA, is currently unknown. In summary, our study uncovers a previously unrecognized regulation of the S-phase checkpoint by poly(ADP-ribosyl)ated proteins, which parallels (in early phase) and interconnects (in late phase) Chk1 to the ATR pathway. 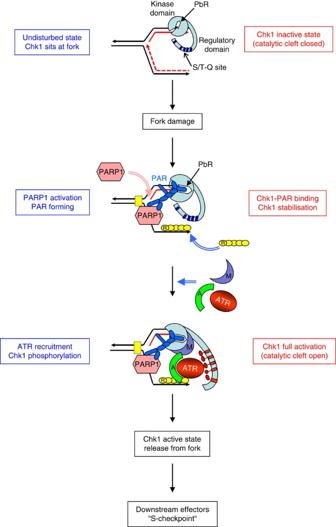Figure 7: A working model of the PAR-mediated Chk1 activation at the replication fork. In the absence of DNA damage, Chk1 is readily associated with the replication fork. The catalytic cleft (regulatory domain) in the C terminus of Chk1 is closed (inactive form) and substrates cannot access the kinase domain. In response to damaged replication forks, PARP1 rapidly binds to the DNA breaks (for example, stalled replication forks) to synthesize PAR onto itself or other acceptor proteins. Chk1 interacts with PAR, supplied by PARP1 (or other poly(ADP-ribosyl)ated proteins), through its N-terminal PbR motif. Single-stranded DNA is coated by RPA (R), which recruits the 9–1–1 complex, TopBP1 (not indicated) and ATR, as well as adaptors (A) and other essential mediators (M) for Chk1, for example, Claspin. In the vicinity of Chk1, which is stabilized by PAR binding, ATR phosphorylates S/T-Q sites within the Chk1 C terminus. PAR binding to Chk1, stabilizes them at the replication forks until full phosphorylation (activation) is achieved, followed by the release of Chk1 from the replication forks. The activation of Chk1 then transduces the damage signal to its downstream effectors that are involved in the S-phase checkpoint. Figure 7: A working model of the PAR-mediated Chk1 activation at the replication fork. In the absence of DNA damage, Chk1 is readily associated with the replication fork. The catalytic cleft (regulatory domain) in the C terminus of Chk1 is closed (inactive form) and substrates cannot access the kinase domain. In response to damaged replication forks, PARP1 rapidly binds to the DNA breaks (for example, stalled replication forks) to synthesize PAR onto itself or other acceptor proteins. Chk1 interacts with PAR, supplied by PARP1 (or other poly(ADP-ribosyl)ated proteins), through its N-terminal PbR motif. Single-stranded DNA is coated by RPA (R), which recruits the 9–1–1 complex, TopBP1 (not indicated) and ATR, as well as adaptors (A) and other essential mediators (M) for Chk1, for example, Claspin. In the vicinity of Chk1, which is stabilized by PAR binding, ATR phosphorylates S/T-Q sites within the Chk1 C terminus. PAR binding to Chk1, stabilizes them at the replication forks until full phosphorylation (activation) is achieved, followed by the release of Chk1 from the replication forks. The activation of Chk1 then transduces the damage signal to its downstream effectors that are involved in the S-phase checkpoint. Full size image Cell culture and DNA damage treatments Primary MEFs were isolated from intercrosses of PARP1 +/− or PARG 110 +/− mice of the 129/Sv background and cultured [64] . All experiments were performed in duplicate and repeated at least twice. 3T3 wild type (A19), PARG 110 −/− , PARP1 −/− (A11) [64] and reconstituted A11 with human PARP1 cDNA (A11/WT2) [42] MEFs were used. Atr f/f CreER T2 MEFs were isolated from E13.5 Atr -floxed embryos [65] . To delete Atr, 2 μM 4-OHT was added to cultures of Atr f/f MEFs for 3 days. These cells were then exposed to various DNA damage agents: 2 μM MNNG (3 h), 10 μM H 2 O 2 (30 min), 4 mM HU (3 h) and 100 J m −2 UV light. COS7, U2OS, HEK293 and MEF cells were cultured and maintained with complete DMEM with 10% fetal calf serum. Cells were exposed to UV (254 nm wavelength in an ultraviolet Stratalinker 2400, Stratagene, Waldbronn, Germany), or incubated with complete medium containing HU (Sigma-Aldrich, Munich, Germany) or MNNG (ABCR GmbH, Karlsruhe, Germany) at the indicated dose and time. Chk1 expression vectors and recombinant protein production The wild-type mouse Chk1 cDNA (wtChk1) was amplified by PCR and inserted into pcDNA4-myc/His (Invitrogen, Darmstadt, Germany). The PbR C/A Chk1 mutation was generated from wtChk1-myc/His as the template using Stratagene’s QuickChange multi site-directed mutagenesis kit according to the manufacturer’s manual. The wtChk1 or PbR C/A Chk1 fragments were subcloned into three different destination vectors: pEGFP-N2 (Clontech, Mountain View, CA, USA); pPuroMaRXf-IV (a kind gift from M.E. Lleonart, Barcelona, Spain); modified pcDNA3-Flag to produce the following vectors: empty GFP (EV-GFP), wtChk1-GFP, PbR C/A Chk1-GFP, Flag-wtChk1, Flag-PbR C/A Chk1, HA-wtChk1, HA-PbR C/A Chk1. Recombinant GST-wtChk1 (14–346, Millipore, Billerica, MA, USA) and GST-PbR C/A Chk1 (GenScript, Aachen, Germany) were purchased. Protein purity was confirmed by SDS–polyacrylamide gel electrophoresis (PAGE) after staining with Coomassie solution (Bio-Rad, Munich, Germany). Transfection and establishment of stable cell lines For interaction studies in vivo , Flag-and HA-tagged vectors were transiently transfected into U2OS or HEK293 cells using Lipofectamine 2000 (Invitrogen) and poly-ethylenimine (Sigma), respectively, according to the manufacturer’s protocol. For the generation of stable cell lines, LinXA packaging cells (a kind gift from M.E. Lleonart) were used to produce retrovirus. Briefly, semiconfluent LinXA cells were transfected with GFP-tagged vectors (30 μg per 10-cm dish) using the calcium phosphate method and retrovirus was collected 2 days later. COS7 cells were infected with the viral supernatant and selected with 2 μg ml −1 puromycin (InvivoGen, San Diego, CA, USA). Populations with transgene expression (GFP+) were sorted by a BD FACS Aria IIu cell sorter (Becton Dickinson, Heidelberg, Germany). Chk1 knockdown For specific siRNA Chk1 knockdown in monkey COS7 cells, four sets of human Chk1 siRNA oligos (1: 5′-CAAGAUGUGUGGUACUUUA-3′; 2: 5′-GAGAAGGCAAUAUCCAAUA-3′; 3: 5′-CCACAUGUCCUGAUCAUAU-3′; 4: 5′-GAAGUUGGGCUAUCAAUGG-3′; Dharmacon, Schwerte, Germany) were used to transfect COS7 cells containing GFP-tagged vectors using Lipofectamine RNAiMAX (Invitrogen) together with Opti-MEM (Gibco, Grand Island, NY, USA) according to the manufacturer’s protocol. For the colony formation assay, siRNA knockdown was performed 2 days before cell plating. To knockdown Chk1 in mouse cells, shChk1-GFP and shLuciferase-GFP (control) vectors [66] were transfected into 3T3 MEFs using Amaxa Nucleofector kit-V (Invitrogen) according to the manufacturer’s protocol. After 2 days, these cells were subjected to the analysis of damage-induced p-Chk1 focus formation by confocal microscopy and of the knockdown efficiency of Chk1 by western blotting. Cell survival assays For the colony formation assay, cells at a density of 3,000 per 10-cm dish were cultured overnight and treated with the indicated doses of HU or MNNG for 3–6 h. Colonies were counted after 10 days (for MEFs) or 7 days (for COS7) after plating. Two short-term cell viability assays were performed. For cell death analysis, COS7 cells stably integrated with GFP-tagged vectors were incubated with siChk1 for 3 days and treated with 1.25 mM HU for 48 h. Harvested cells were stained with Annexin V-APC antibody (1:100; 550475, BD Pharmingen, Heidelberg, Germany) and subjected to flow cytometric analysis. For cell survival counting, COS7 cells stably expressing GFP-tagged vectors were cultured in 96-well dishes (750 cells per well) for 24 h, subsequently followed by transfection with Chk1 siRNA or nt-siRNA. After 54 h, cells were treated with 1.25 mM HU for 20 h and cultured for an additional 20 h in HU-free medium before fixation. Nuclei were stained with 4′,6-diamidino-2-phenylindole and counted by high-content analysis microscopy (Cellomics Arrayscan V TI , Thermo Scientific, Pittsburgh, PA, USA). Each experiment was repeated at least twice. RDS assay MEF cells were plated at a density of 3.3 × 10 4 per well of a six-well plate and cultured in complete DMEM for 5 h at 37 °C. UCN-01 (100 nM; Sigma-Aldrich) was added 18 h before assaying. COS7 cells stably transfected with various GFP-tagged vectors were transfected with either siChk1 or control (nt-Chk1) oligos 3 days before the RDS assay. These cells were incubated with 0.05 μCi ml −1 14 C-thymidine (Hartmann Analytic, Braunschweig, Germany) for 18 h at 37 °C, before treatment with 3 J m −2 UV light. Cells were labelled with medium containing 1 μCi ml −1 3 H-thymidine (Hartmann Analytic) for 3 h. Following solubilization in 0.3 N NaOH, the radioactivity in cell lysates was counted using a Liquid Scintillation Analyzer Tri-Carb 2800 TR (PerkinElmer, Rodgau, Germany). The DNA synthesis ratio ( 3 H/ 14 C) was calculated. IP and immunoblotting MEFs with or without pre-incubation (1 h) with 10 μM PARP inhibitor (PJ-34) were treated with or without 2 or 4 mM HU for 3 h and harvested by scraping cells on ice, and then washed with cold PBS containing 25 μM PARG inhibitor (GPI18214, MGI Pharma, Bloomington, MN, USA). HEK293 cells were co-transfected with Flag-Claspin (Addgene, Cambridge, MA, USA) and HA-Chk1 (wtChk1 or PbR C/A Chk1), or HA-BRCA1 (Addgene) and Flag-Chk1 (wtChk1 or PbR C/A Chk1) plasmids. Two days after transfection, these cells were treated with 4 mM HU for 3 h before harvest. Cell pellets were lysed in cold lysis buffer containing 50 mM Tris–HCl pH 7.4, 150 mM NaCl, 1% NP40, 1 mM EDTA, 1 mM phenylmethylsulphonyl fluoride, 1 mM Na 3 VO 4 , 10 mM NaF, 25 μM PARG inhibitor, 1 × Complete Protease Inhibitor Cocktail (Roche, Mannheim, Germany) and 1 × PhosSTOP phosphatase inhibitor cocktail (Roche). After centrifugation, the supernatants were used for Co-IP. To prevent the interference of the IgG bands in Co-IP, TrueBlot IP beads (eBioscience, San Diego, CA, USA) and Clean-Blot IP detection reagent (Thermo Scientific, Rockford, IL, USA) were used according to the manufacturers’ manual. Cell lysates and immunoprecipitates were subjected to either nitrocellulose membranes (for non-denaturing slot-blot) or separation on SDS–PAGE gels (polyvinylidene fluoride) for antibody blotting. To analyse the interaction of PAR with Chk1 or with p-Chk1 in Atr-deficient conditions by Co-IP and non-denaturing slot-blot assays, 10 μM ATR inhibitor (ETP-46464, a kind gift from Dr Fernandez-Capetillo) was used as described previously [49] . The following antibodies were used: p-Chk1 (S317) (1:1,000 dilution; A300-163 A, Bethyl Laboratories, Montgomery, TX, USA), Chk1 (1:1,000; A300-161 A; Bethyl Laboratories and 1:500; ab16130, Abcam, Cambridge, UK), p-Cdc25a (S75) (1:1,000; ab47279, Abcam), PAR (1:1,000; LP98-10; Enzo Life Sciences, Lörrach, Germany), PARP1 (1:1,000; C2-10, Trevigen, Gaithersburg, MD, USA and 1:1,000; N20, Santa Cruz Biotechnology, Santa Cruz, CA, USA), ATR (1:1,000; NB100-323, Novus Biological, Cambridge, UK), ATM (1:500; NB100-309, Novus Biological), p-ATM (S1981) (1:1,000; 200-301-400, Rockland), GST (1:1,000; sc-138, Santa Cruz Biotechnology), Flag-tag (1:1,000, F1804, Sigma-Aldrich), HA-tag (1:10000, A190-208 A, Bethyl laboratories) and β-actin (1:10,000; A5441, Sigma-Aldrich). Full-length images of IBs are shown in Supplementary Fig. S8 . Immunofluorescence analysis of cells For DNA damage-induced focus formation, 3T3 MEFs were treated with 4 mM HU for 5 h or 10 J m −2 UV light. To label S-phase cells, cells were incubated with 2 μg ml −1 EdU (Invitrogen) using Click-iT kit (conjugated with EdU-Cy5; Invitrogen) for 1 h before DNA damage treatment. To visualize the foci, cells were fixed in 3.7% formaldehyde, 0.1% Triton X-100 in PBS and incubated with primary antibodies in PBS/7% BSA at 4 °C overnight. The following primary antibodies were used: PAR (1:200; 10 H; Enzo Life Sciences) and p-Chk1 (S317) (1:200; A300-163 A; Bethyl Laboratories). For indirect immunofluorescence detection, the following secondary antibodies were used: anti-mouse-FITC (1:400; F2883; Sigma-Aldrich) and anti-rabbit-Cy3 (1:400; C2306; Sigma-Aldrich). The specimens were mounted in Prolong Gold antifade reagent with 4′,6-diamidino-2-phenylindole (Invitrogen) and visualized under an Axio Imager Apotome microscope (Zeiss, Jena, Germany). The camera (MRM Axiocam, Zeiss) and the structured illumination were controlled by the Axiovision software (Zeiss). To collect full information of the spot fluorescence (focus), Z-stacks containing 15 optical layers were recorded every 250 nm. Cells containing more than five foci were counted as foci positive. At least 200 cells were analysed for each treatment. Each experiment was repeated at least twice. After transfecting the shChk1-GFP or the shLuciferase vector into 3T3 MEF cells, GFP-positive cells were visualized by the GFP-booster kit (Chromotek, Planegg-Martinsried, Germany) in combination with EdU-labelling (as described above). Isolation of proteins from nascent chromatin (iPOND) assay The iPOND assay was performed essentially as described [47] . Briefly, HEK293 cells or MEF cells were plated to 140 mm dishes 2 days before the experiment. Cells (10 8 HEK cells or 4 × 10 8 MEF cells per sample) were pulse labelled with 10 μM EdU for 10 min. For the pulse-chase experiment, the EdU was replaced with media containing 10 μM thymidine for 30 min. After 3 mM HU treatment of indicated times, cells were cross-linked in 1% formaldehyde in PBS for 20 min and quenched with 0.125 M glycine. Cell pellets were suspended in 0.25% Triton X-100 in PBS, washed once with 0.5% BSA in PBS and once with PBS. Cells were incubated in click reaction buffer (2 mM CuSO 4 , 10 μM biotin azide (Invitrogen) and 10 mM sodium ascorbate) for 2 h at a concentration of 1 × 10 8 cells per 5 ml. Cell pellets were washed once with 0.5% BSA/PBS and once with PBS before suspension in lysis buffer (1% SDS, 50 mM Tris (pH 8.0)), 1 × Complete Protease Inhibitor Cocktail (Roche), 1 × PhosphoSTOP (Roche) and sonication. Samples were centrifuged, filtered through a 90-μm nylon mesh, and diluted 1:1 with PBS containing 1 × Complete Protease Inhibitor Cocktail (Roche) and 1 × PhosphoSTOP (Roche). Streptavidin agarose resin (Millipore) (50 μl resin per 10 8 cells) was incubated with the samples and rotated for 20 h at 4 °C. Captured proteins were eluted and cross-links were reversed in 2 × Laemmli buffer (4% SDS, 20% glycerol, 125 mM Tris pH 6.8, 0.1% (w/v) bromophenol blue and 0.2 M dithiothreitol (DTT)) by incubating for 25 min at 95 °C. Proteins were resolved on SDS–PAGE and detected by western blotting. All solutions starting from the fixation buffer were supplemented with 0.5 mM Na 3 VO 4 , 2.5 mM NaF, 1 mM β-glycerophosphate, 1 μM PARP inhibitor AG014699 (Pfizer, New York, USA) and 25 μM PARG inhibitor GPI18214 (MGI Pharma). Synthesis and fractionation of PAR PAR was synthesized, purified and HPLC fractionated as described [52] , [67] , [68] . Briefly, a reaction mixture containing 150 nM recombinant PARP1 was incubated in 100 mM Tris–HCl pH 7.8, 10 mM MgCl 2 , 10 mM DTT, 60 μg ml −1 histone H1, 60 μg ml −1 histone type IIa, 1 mM NAD + and 50 μg ml −1 double-stranded activator oligonucleotide 5′-GGAATTCC-3′ for 15 min at 37 °C. The reaction was stopped in a final concentration of 10% (v/v) trichloroacetic acid (TCA) followed by ethanol precipitation. PAR was detached from proteins by 0.5 M KOH/50 mM EDTA treatment followed by phenol-chloroform-isoamyl-alcohol purification. An aqueous solution of PAR was HPLC-fractionated consulting a DNA Pac PA100 anion-exchange column (DIONEX) using a NaCl gradient. Modified sequencing gels for PAR quality check were carried out as described [69] using GELCODE Color silver stain (Pierce, Thermo-Fisher Scientific, Bonn, Germany). PAR-binding assay Proteins (1 pmol) were spotted onto a nitrocellulose membrane. The synthesis and purification of radioactively labelled PAR and the analysis of PAR binding to proteins were performed as described previously [32] . The membrane was washed with TBS-T buffer containing 600 mM NaCl and 20 mM EDTA. PAR bound to spotted protein was detected by autoradiography and protein loading was confirmed by immunoblotting. Three independent experiments were performed. Chk1 in vitro activity assay Kinase assay was performed as described previously [70] . Briefly, indicated amounts of recombinant GST-Chk1 proteins were incubated with size-fractionated PAR (26–30 moieties=short; >65 moieties=long) or 1 μM Chk1 inhibitor UCN-01 for 30 min on ice and the kinase reaction (30 min, 30 °C) was initiated by the addition of kinase buffer (final concentration: 25 mM Tris pH 7.5, 5 mM MgCl 2 , 0.5 mM DTT, 5 mM ATP). Each reaction contained 10 μCi [γ- 32 P]-ATP and 2 μg GST-Cdc25a (101–140) [70] . Reactions were stopped by the addition of SDS–PAGE loading buffer, proteins were separated by SDS–PAGE, blotted onto polyvinylidene fluoride membranes and radioactive labelling was detected by autoradiography. Loading and protein modifications were detected by immunoblotting with indicated antibodies. Three independent experiments were performed. Poly(ADP-ribosyl)ation of PARP1 and Chk1 kinase assay PAR synthesis was performed at 37 °C for 90 min using 10 units recombinant PARP1 (Trevigen, 4668-100-01, Gaithersburg, Maryland, USA) with 1 × activated DNA (Trevigen) and 200 μM NAD + in 50 mM Tris pH 8.0, 50 mM NaCl and 5 mM MgCl 2 . The reaction was stopped by addition of 1 μM PARP inhibitor AG014699. The reaction product was added to GST-Chk1 to carry out the in vitro kinase assay as described above. How to cite this article: Min, W. et al. Poly(ADP-ribose) binding to Chk1 at stalled replication forks is required for S-phase checkpoint activation. Nat. Commun. 4:2993 doi: 10.1038/ncomms3993 (2013).